TRF1 is a stem cell marker and is essential for the generation of induced pluripotent stem cells TRF1 is a component of the shelterin complex that protects chromosome ends. TRF1 deficiency leads to early embryonic lethality and to severe organ atrophy when deleted in adult tissues. Here we generate a reporter mouse carrying a knock-in eGFP-TRF1 fusion allele to study the role of TRF1 in stem cell biology and tissue homeostasis. We find that eGFP–TRF1 expression in mice is maximal in known adult stem cell compartments and show that TRF1 ensures their functionality. eGFP–TRF1 is highly expressed in induced pluripotent stem cells, uncoupled from the telomere elongation associated with reprogramming. Selection of eGFP–TRF1-high induced pluripotent stem cells correlates with higher pluripotency as indicated by their ability to form teratomas and chimeras. We further show that TRF1 is necessary for both induction and maintenance of pluripotency, and that TRF1 is a direct transcriptional target of Oct3/4. Telomeres are essential to protect the ends of chromosomes from degradation and DNA repair activities, thus ensuring chromosome stability [1] . Vertebrate telomeres are composed of tandem repeats of the TTAGGG sequence bound by a six-protein complex known as shelterin [2] . Shelterin encompasses TRF1, TRF2, POT1, TIN2, TPP1 and RAP1. TRF1 binds to double-stranded TTAGGG repeats and its abundance at telomeres is proportional to the length of repeats [2] , [3] , being a potentially good reporter of telomere length in vivo . TRF1 abrogation leads to early embryonic lethality at the blastocyst stage [4] , suggesting an essential role for TRF1 in early mouse development. Conditional TRF1 deletion in adult tissues, including stratified epithelia and bone marrow, leads to severe tissue atrophy and dysfunction, which are coincidental with high levels of telomere damage and, in the case of the bone marrow, with severe telomere shortening [5] , [6] , suggesting that TRF1 may be important for adult stem cell compartments and maintenance of organ homeostasis. Interestingly, TRF1 has been recently identified among the genes that show higher expression levels in embryonic stem (ES) cells and induced pluripotent stem (iPS) cells compared with somatic cells [7] , suggesting a potential role for TRF1 in the acquisition and/or maintenance of pluripotency. In this regard, a number of links between telomere biology and pluripotency have been recently established [8] , [9] , [10] . On one hand, telomerase activity is highly expressed in mouse and human pluripotent ES cells [9] , [11] , [12] . In addition, telomerase is highly upregulated during generation of iPS cells [9] , [13] , [14] , [15] where it is responsible for elongation of telomeres during and post induction of pluripotency to reach the hyper-long telomeres characteristic of pluripotent ES cells [9] , [15] . Telomerase is also essential for the maintenance of chromosome integrity in the resulting iPS cells [8] , [9] . In addition to telomerase, the shelterin protein Tpp1 has been also described to be necessary for telomerase-mediated telomere elongation in iPS cells by bringing telomerase to the telomere. In particular, Tpp1-deficient iPS cells fail to elongate telomeres in spite of normal telomerase expression [10] . To further address the regulation of TRF1 in adult stem cells and pluripotent stem cells, we generated a knock-in (KI) TRF1 allele in which TRF1 is tagged to the enhanced green fluorescent protein (eGFP) reporter protein. In this context, generation of a reporter mouse for TRF1 is a valuable tool not only to understand the regulation of TRF1 expression in normal and pluripotent/adult stem cells, but also to address whether cells with high TRF1 levels are associated with higher stemness/pluripotency. Generation of mice with a KI eGFP–TRF1 allele Mice with a KI eGFP-tag behind the ATG start codon in the first exon of the TRF1 locus were generated ( Fig. 1a ). The neomycin selection cassette was flanked by loxP sites to generate the eGFP–TRF1 allele by using Cre-recombinase. Wild-type and heterozygous eGFP–TRF1 +/KI mice were born at Mendelian ratios and are viable, fertile and show no phenotypes related to TRF1 abrogation, such as hair loss, skin hyperpigmentation or bone marrow aplasia ( Supplementary Fig. S1a–e ) [5] , [6] . However, we failed to obtain mice of the eGFP–TRF1 KI/KI genotype owing to embryonic lethality around day E13.5. In particular, only 6% of E13.5 embryos were eGFP–TRF1 KI/KI versus the 25% expected ratio from eGFP–TRF1 +/KI crosses ( Supplementary Fig. S1a ). Given that full TRF1 ablation leads to embryonic lethality at the blastocyst stage [4] , the observed late embryonic lethality of homozygous eGFP–TRF1 KI/KI mice suggest that the eGFP–TRF1 allele is hypomorphic. In line with this, although eGFP–TRF1 KI/KI mouse embryonic fibroblasts (MEFs) are able to divide in vitro ( Supplementary Fig. S1b,c ), they show decreased proliferation rates and increased senescence-associated β-gal staining compared with wild-type and heterozygous MEFs ( Supplementary Fig. S1b ) [6] , [16] . In addition, eGFP–TRF1 KI/KI MEFs showed slightly augmented frequencies of sister telomere fusions (1–2 sister-chromatid fusions per metaphase, a frequency tenfold lower than that for complete TRF1 abrogation) and similar frequencies of multitelomeric signals related to telomere fragility (MTS) to TRF1 -null MEFs ( Supplementary Fig. S2a,c ) [6] . This degree of telomere dysfunction, however, did not lead to increased DNA damage in eGFP–TRF1 KI/KI MEFs, as indicated by similar frequencies of 53BP1-positive cells and of 53BP1 foci colocalizing to telomeres (telomere-induced foci, or TIFs) in the different genotypes ( Supplementary Fig. S2b ). These findings suggest a largely normal telomere capping function of the eGFP–TRF1 fusion protein, also in agreement with the very low frequencies of end-to-end fusions found in eGFP–TRF1 KI/KI MEFs. 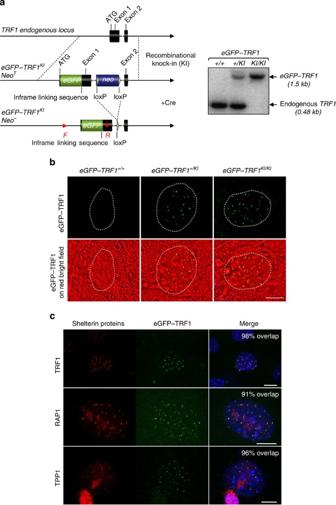Figure 1: eGFP–TRF1 protein is nuclear and localizes to telomeres. (a) Left panel: schematic representation of theeGFP–TRF1allele. Right panel: genotyping of the different alleles by PCR analysis. F/R: forward/reverse primer for PCR analysis, Neo: neomycin cassette. (b) Expression of eGFP–TRF1 fusion protein in livingeGFP–TRF1+/KIandeGFP–TRF1KI/KIMEFs (passage 2) as seen by confocal microscopy. Top panels: eGFP–TRF1 fluorescence; including red contrasted bright field picture on the bottom to determine nuclear localization (nuclei are indicated by dotted line) of the eGFP–TRF1 fusion protein. Scale bar: 10 μm. (c) Colocalization studies between the indicated shelterin proteins and eGFP–TRF1 ineGFP–TRF1+/KIMEFs (passage 2). The percentage of visible colocalization of the indicated shelterin signal with the eGFP–TRF1 signal is indicated. Green, eGFP–TRF1; red, immunostained shelterins with second antibodies labelled with Cy3 or A555 (TPP1). Scale bars, 10 μm. Figure 1: eGFP–TRF1 protein is nuclear and localizes to telomeres. ( a ) Left panel: schematic representation of the eGFP–TRF1 allele. Right panel: genotyping of the different alleles by PCR analysis. F/R: forward/reverse primer for PCR analysis, Neo: neomycin cassette. ( b ) Expression of eGFP–TRF1 fusion protein in living eGFP–TRF1 +/KI and eGFP–TRF1 KI/KI MEFs (passage 2) as seen by confocal microscopy. Top panels: eGFP–TRF1 fluorescence; including red contrasted bright field picture on the bottom to determine nuclear localization (nuclei are indicated by dotted line) of the eGFP–TRF1 fusion protein. Scale bar: 10 μm. ( c ) Colocalization studies between the indicated shelterin proteins and eGFP–TRF1 in eGFP–TRF1 +/KI MEFs (passage 2). The percentage of visible colocalization of the indicated shelterin signal with the eGFP–TRF1 signal is indicated. Green, eGFP–TRF1; red, immunostained shelterins with second antibodies labelled with Cy3 or A555 (TPP1). Scale bars, 10 μm. Full size image The eGFP–TRF1 fusion protein tracks telomeres in vivo Next, we determined whether the expression of the eGFP–TRF1 fusion protein was nuclear and colocalized with telomeres. We detected eGFP expression at the nuclei of living MEFs by using confocal microscopy in both heterozygous- and homozygous-KI cells but not in wild-type cells ( Fig. 1b ). Furthermore, eGFP signals showed a >90% colocalization with endogenous TRF1, RAP1 and TPP1 shelterin proteins in eGFP–TRF1 +/KI MEFs ( Fig. 1c ) (see Methods). Thus, the eGFP–TRF1 fusion protein is nuclear and localizes to telomeres, representing a new tool to track TRF1 and telomeres in vivo by using direct fluorescence. eGFP–TRF1 expression marks adult stem cell compartments We previously reported that the cells harbouring the longest telomeres within a tissue are enriched at the known stem cell compartments, while cells showing the shortest telomeres are located at the more differentiated compartments [17] . Here, we set to address whether TRF1 expression showed a similar distribution to that of telomere length in the skin and small intestine adult stem cell compartments. To this end, we followed eGFP expression in both skin and small intestine from eGFP–TRF1 +/KI mice. In the case of telogen tail-skin hair follicles, we found maximum eGFP fluorescence at the known stem cell compartments of the epidermis (EP), sebaceous gland (SG) and the middle hair follicle bulge [18] , [19] , [20] , [21] , [22] , [23] , while eGFP fluorescence was lowest at the interfollicular EP ( Fig. 2a–c ). Moreover, eGFP–TRF1 fluorescence was higher in CK15-positive cells compared with CK15-negative cells, a bona fide marker of hair bulge stem cells [24] ( Fig. 2d ), in agreement with previous findings for telomere length [17] . Interestingly, eGFP–TRF1 fluorescence decreased by 72.5% from the stem cell compartments to interfollicular EP ( Fig. 2b ), suggesting that TRF1 expression is downregulated associated with tissue differentiation. 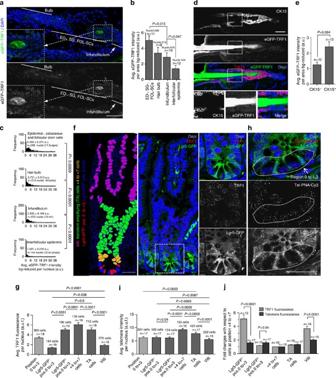Figure 2: TRF1 levels are highest in adult stem cell compartments of the skin and the small intestine. (a) Representative image of eGFP–TRF1 fluorescence in different compartments of tail-skin follicles (telogen) ofeGFP–TRF1+/KImice. eGFP–TRF1 intensity decreases from the putative stem cell niches towards the more differentiated compartments (interfollicular skin). (b,c) eGFP–TRF1 fluorescence quantification in the EP-, SG-, follicular (FOL) stem cells, bulb, infundibulum and interfollicular areas.n, independent follicles (b). Error bars: s.e.m. Statistical analysis: two-sided Student’st-tests. Scale bar, 50 μm. (d) Representative image of a Cytokeratin15 (CK15)-stained telogen tail-skin hair follicle (top); middle: eGFP–TRF1 fluorescence and merge. Close-up shows CK15-positive and -negative cells. Scale bar, 50 μm. (e) Quantification of background (bg)-corrected eGFP–TRF1 fluorescence in CK15-positive and -negative cells.n, independent follicles;N=3 mice. Error bars: s.e.m. Statistical analysis: two-sided Student’st-tests. (f) Left panel: cell type definition, using the indicated colour code. Right panels: Lgr5-eGFP fluorescence (green; bottom close-up), TRF1 fluorescence (red; middle close-up) and merge (top close-up) in small intestine crypt/villi of a heterozygousLgr5-eGFPintestine. Scale bar, 50 μm. (g) Average TRF1 fluorescence per nucleus in arbitrary units of fluorescence (a.u.f.). Highest expression of TRF1 is seen in +4 to +7 cells followed by Lgr5-GFP+and TA cells. Lgr5-GFP+cells in the crypt express much higher levels of TRF1 than neighbouring, Lgr5-GFP−Paneth cells.n, independent crypts;N=4 mice. Error bars: s.e.m. Statistical analysis: two-tailed, paired (within crypts)t-test. (h) Representative picture of a GFP-telomere immuno-FISH. Bottom: Lgr5-GFP fluorescence marks Lgr5+ cells. Tel-PNA-Cy3 probe labels telomere. Top: merge, showing similar telomere intensities in Lgr5+and Lgr5−cells in the 0 to +3 compartment. Scale bar, 10 μm. (i) Nuclear telomere intensity per nucleus (correlates with telomere length). No differences are observed in Lgr5-GFP−cells and Lgr5-GFP+cells in the 0 to +3 region.n, independent crypts;N=3 mice. Error bars: s.e.m. Statistical analysis: two-tailed paired (within crypts)t-test. (j) Fold changes of TRF1 levels versus telomere length in different villi/crypt compartments. Numbers fromgandh. Error bars: s.e.m. Statistical analysis: two-sided Student’st-test. Figure 2: TRF1 levels are highest in adult stem cell compartments of the skin and the small intestine. ( a ) Representative image of eGFP–TRF1 fluorescence in different compartments of tail-skin follicles (telogen) of eGFP–TRF1 +/KI mice. eGFP–TRF1 intensity decreases from the putative stem cell niches towards the more differentiated compartments (interfollicular skin). ( b , c ) eGFP–TRF1 fluorescence quantification in the EP-, SG-, follicular (FOL) stem cells, bulb, infundibulum and interfollicular areas. n , independent follicles ( b ). Error bars: s.e.m. Statistical analysis: two-sided Student’s t- tests. Scale bar, 50 μm. ( d ) Representative image of a Cytokeratin15 (CK15)-stained telogen tail-skin hair follicle (top); middle: eGFP–TRF1 fluorescence and merge. Close-up shows CK15-positive and -negative cells. Scale bar, 50 μm. ( e ) Quantification of background (bg)-corrected eGFP–TRF1 fluorescence in CK15-positive and -negative cells. n , independent follicles; N =3 mice. Error bars: s.e.m. Statistical analysis: two-sided Student’s t- tests. ( f ) Left panel: cell type definition, using the indicated colour code. Right panels: Lgr5-eGFP fluorescence (green; bottom close-up), TRF1 fluorescence (red; middle close-up) and merge (top close-up) in small intestine crypt/villi of a heterozygous Lgr5-eGFP intestine. Scale bar, 50 μm. ( g ) Average TRF1 fluorescence per nucleus in arbitrary units of fluorescence (a.u.f.). Highest expression of TRF1 is seen in +4 to +7 cells followed by Lgr5-GFP + and TA cells. Lgr5-GFP + cells in the crypt express much higher levels of TRF1 than neighbouring, Lgr5-GFP − Paneth cells. n , independent crypts; N =4 mice. Error bars: s.e.m. Statistical analysis: two-tailed, paired (within crypts) t- test. ( h ) Representative picture of a GFP-telomere immuno-FISH. Bottom: Lgr5-GFP fluorescence marks Lgr5+ cells. Tel-PNA-Cy3 probe labels telomere. Top: merge, showing similar telomere intensities in Lgr5 + and Lgr5 − cells in the 0 to +3 compartment. Scale bar, 10 μm. ( i ) Nuclear telomere intensity per nucleus (correlates with telomere length). No differences are observed in Lgr5-GFP − cells and Lgr5-GFP + cells in the 0 to +3 region. n , independent crypts; N =3 mice. Error bars: s.e.m. Statistical analysis: two-tailed paired (within crypts) t -test. ( j ) Fold changes of TRF1 levels versus telomere length in different villi/crypt compartments. Numbers from g and h . Error bars: s.e.m. Statistical analysis: two-sided Student’s t -test. Full size image In the case of back skin hair follicles in anagen (9 days after plucking; Methods), we found the highest percentage of eGFP–TRF1-expressing cells and the strongest eGFP–TRF1 signal at the junctional zone that contains the epidermal-, SG- and follicular stem cells, followed by the outer root sheath (migrating progenitor cells) and the hair matrix, where cycling progenitors and transient amplifying cells reside ( Supplementary Fig. S3a–c ). The differentiated cells at the inner root sheath did not show detectable eGFP–TRF1 signal whereas the infundibulum showed heterogeneity in eGFP signal ( Supplementary Fig. 3a–c ). Interestingly, the cycling cells of the hair matrix express lower eGFP–TRF1 levels than the lower cycling junction zone cells, suggesting that eGFP–TRF1 levels do not correlate with proliferation indexes. Next, we studied eGFP–TRF1 expression at small intestine epithelium. We found the highest eGFP fluorescence in the area above the region containing paneth cells (position 0 to +3), namely from cellular position +4 to +7, and the lowest expression at the villi ( Supplementary Fig. S4a–c ). Again, eGFP–TRF1 expression decreased by 94% from the less differentiated +4 to +7 positions to the more differentiated villi cells ( Supplementary Fig. S5a,b,d ). In a similar manner, the endogenous TRF1 protein was decreased by 80% from positions +4 to +7 to villi cells ( Supplementary Fig. S5a,c,e ), indicating a similar behaviour of both the eGFP–TRF1 fusion protein and the endogenous TRF1 with differentiation. Recent reports indicate that small intestine stem cells are interspersed with differentiated cells at the 0 to +3 region, and can be identified by high Lgr5 expression and presence of long telomeres [25] , [26] . To address whether Lgr5+ cells show high TRF1 expression compared with Lgr5-negative Paneth cells, we determined TRF1 fluorescence in Lgr5-eGFP reporter mice [27] . Interestingly, TRF1 expression was not homogeneous at the Paneth region, with the eGFP-Lgr5-positive cells (Lgr5+) showing high TRF1 expression compared with the eGFP-negative (Lgr5–) cells ( Fig. 2f ). Unexpectedly, telomere length at position 0 to +3 was similar in eGFP-Lgr5-positive cells and eGFP-negative cells, being significantly lower than that of cells at +4 to +7 positions ( Fig. 2h ). These results are in agreement with our previous findings, mapping the longest telomeres to the +4 to +7 position [17] , and indicate uncoupling between TRF1 levels and telomere length. Also in line with this notion, the fold change in TRF1 expression from the less differentiated +4 to +7 cells to the more differentiated Lgr5-eGFP-negative and villi cells was significantly more pronounced than for telomere length ( Fig. 2j ). Together, these findings demonstrate a previously unnoticed enrichment of TRF1 expression at the adult stem cell compartments of the skin and the small intestine. Finally, the presence of longer telomeres at the +4 to +7 compared with the Lgr5+ cells may suggest the existence of additional stem cells at the +4 to +7 position with longer telomeres than the Lgr5-positive cells, in line with recent findings suggesting that Lgr5-positive cells are dispensable for intestine homeostasis [28] . Intestinal TRF1 ablation leads to severe GI atrophy To address whether TRF1 expression in adult stem cell compartments is important for tissue homeostasis, we conditionally deleted TRF1 in the small intestine by crossing TRF1 lox/lox mice generated by us [6] with Villin-CreERT2 mice [29] , thus targeting TRF1 deletion to villin-expressing tissues [30] , [31] , [32] . By using PCR, we detected specific excision of TRF1 in the villin-expressing tissues, such as the small intestine and colon but not the spleen ( Supplementary Fig. S6a ). As control, TRF1 +/+ ; Villin-CreERT2 +/T mice showed normal small intestine morphology and enriched TRF1 expression at the crypts, particularly at the +4 to +7 position ( Fig. 3a , upper panel; Fig. 3g ; Supplementary Fig. S6b , upper panel). Interestingly, TRF1 lox/lox ; Villin-CreERT2 +/T mice showed a dramatic decrease of TRF1 expression in most intestinal cells ( Supplementary Fig. S6b , bottom panel; Fig. 3g ), concomitant with severe weight loss of viability in some mice ( Supplementary Fig. S6c ) and aberrant intestinal morphology going from moderate to severe lesions ( Fig. 3a ). Moderate lesions showed shortening of the villi and a diffuse inflammatory infiltration with lymphoid cells ( Fig. 3a , middle panels), as well as decreased crypt/villi density ( Fig. 3b ). In the severe lesions, the morphology of the intestine was lost, showing severely atrophic microvilli, a higher amount of lymphoid infiltrates and a lamina propia in the duodenum without Brunners glands ( Fig. 3a , bottom panels). This was coincidental with an increased abundance of apoptotic cells and cells with big, endoreduplicated nuclei ( Fig. 3c ; quantification in Fig. 3d ). Increased apoptosis was also confirmed by caspase3-positive staining ( Supplementary Fig. S7a,b ). Interestingly, the highest amount of apoptotic and endoreduplicated cells was found at the stem cell region from +4 to +7 positions ( Fig. 3d ). 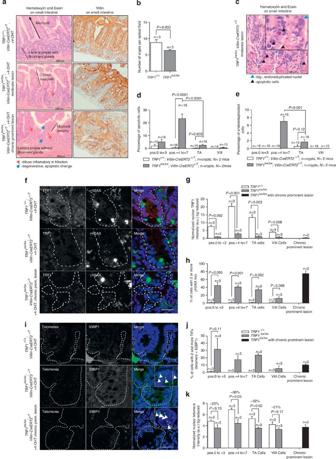Figure 3: Conditional TRF1 deletion in the small intestine. (a) Haematoxylin and eosin (H&E) staining and Villin immunostaining ofTRF1+/+;Villin-CreERT2+/TandTRF1lox/lox;Villin-CreERT2+/Tintestines treated with 4-OHT showing moderate and severe chronic prominent lesions. Treated intestines show shortened villi without columnar absorptive cells (middle and lower pictures). In severe cases, the epithelial lining is lost and a chronic inflammatory response is seen in mucosa and lamina propria (bottom pictures). (b) The number of crypts per optical field is significantly decreased inTRF1lox/lox; Villin-CreERT2+/Tintestines compared with theTRF1+/+mice. Indicated: number of crypts by × 200 magnification, aligned parallel to the picture border.n, different intestines. Error bars: s.e.m. Statistical analysis: two-sided Student’st-test. (c) Representative H&E image showing apoptotic and endoreduplicated nuclei inTRF1lox/lox;Villin-CreERT2+/Tintestines upon 4-OHT treatment (black arrows: apoptosis; blue arrow: endoreduplication). (d,e) Percentage of apoptotic and endoreduplicated cells in the indicated crypt compartments. The highest numbers are found at positions +4 to +7, which contain a putative stem cell population. Error bars: s.e.m. Statistical analysis: two-sided Student’st-test. (f) Representative γH2AX and TRF1 immunofluorescence pictures ofTRF1lox/lox;Villin-CreERT2+/TandTRF1+/+;Villin-CreERT2+/Tintestines. In intestines with a chronic, atrophic structure, compartments were indistinguishable. TRF1 foci intensity in theTRF1lox/lox;Villin-CreERT2+/Tmice is significantly decreased. Scale bar, 50 μm. (g,h) Graphs of background (bg)-reduced TRF1 intensities (arbitrary units (a.u.)) per nucleus and percentages of cells in the indicated compartments showing two or more γH2AX foci per nucleus. Almost no TRF1 foci are detected in intestines with atrophic structures with chronic permanent lesions.n, different intestines. Error bars: s.e.m. Statistical analysis: two-sided Student’st-test. (i) Representative pictures of a 53BP1 immuno-telomere Q-FISH on intestines. Scale bar, 50 μm. (j,k) Cells with two or more TIF (telomeres positive for 53BP1). In wild-type conditions, TIFs are rare, avoiding statistical comparison (j). Background-corrected telomere intensities per nucleus. All intestinal compartments decreased in telomere length, most pronounced at positions +4 to +7 (k).n, different intestines. Error bars: s.e.m. Statistical analysis: two-sided Student’st-test. Figure 3: Conditional TRF1 deletion in the small intestine. ( a ) Haematoxylin and eosin (H&E) staining and Villin immunostaining of TRF1 +/+ ;Villin-CreERT2 +/T and TRF1 lox/lox ;Villin-CreERT2 +/T intestines treated with 4-OHT showing moderate and severe chronic prominent lesions. Treated intestines show shortened villi without columnar absorptive cells (middle and lower pictures). In severe cases, the epithelial lining is lost and a chronic inflammatory response is seen in mucosa and lamina propria (bottom pictures). ( b ) The number of crypts per optical field is significantly decreased in TRF1 lox/lox ; Villin-CreERT2 +/T intestines compared with the TRF1 +/+ mice. Indicated: number of crypts by × 200 magnification, aligned parallel to the picture border. n , different intestines. Error bars: s.e.m. Statistical analysis: two-sided Student’s t- test. ( c ) Representative H&E image showing apoptotic and endoreduplicated nuclei in TRF1 lox/lox ;Villin-CreERT2 +/T intestines upon 4-OHT treatment (black arrows: apoptosis; blue arrow: endoreduplication). ( d , e ) Percentage of apoptotic and endoreduplicated cells in the indicated crypt compartments. The highest numbers are found at positions +4 to +7, which contain a putative stem cell population. Error bars: s.e.m. Statistical analysis: two-sided Student’s t- test. ( f ) Representative γH2AX and TRF1 immunofluorescence pictures of TRF1 lox/lox ;Villin-CreERT2 +/T and TRF1 +/+ ;Villin-CreERT2 +/T intestines. In intestines with a chronic, atrophic structure, compartments were indistinguishable. TRF1 foci intensity in the TRF1 lox/lox ;Villin-CreERT2 +/T mice is significantly decreased. Scale bar, 50 μm. ( g , h ) Graphs of background (bg)-reduced TRF1 intensities (arbitrary units (a.u.)) per nucleus and percentages of cells in the indicated compartments showing two or more γH2AX foci per nucleus. Almost no TRF1 foci are detected in intestines with atrophic structures with chronic permanent lesions. n , different intestines. Error bars: s.e.m. Statistical analysis: two-sided Student’s t- test. ( i ) Representative pictures of a 53BP1 immuno-telomere Q-FISH on intestines. Scale bar, 50 μm. ( j , k ) Cells with two or more TIF (telomeres positive for 53BP1). In wild-type conditions, TIFs are rare, avoiding statistical comparison ( j ). Background-corrected telomere intensities per nucleus. All intestinal compartments decreased in telomere length, most pronounced at positions +4 to +7 ( k ). n , different intestines. Error bars: s.e.m. Statistical analysis: two-sided Student’s t- test. Full size image In agreement with the known role for TRF1 in telomere protection [6] , we found increased numbers of γH2AX-positive cells in all intestinal compartments, with the highest abundance in the severe lesions ( Fig. 3f ). In addition, TIF, which represent telomeres colocalizing with DNA damage foci, were also increased upon TRF1 ablation ( Fig. 3i ). Of note, although DNA damage was found at all intestinal compartments, the fact that apoptotic and endoreduplicated cells were preferentially found at the positions +4 to +7 and to as lesser extend in the TA compartment suggests that the less differentiated compartments show higher sensitivity to the DDR induced by TRF1 ablation. Finally, we observed that TRF1 deletion led to a significant shortening of telomeres in all the intestinal compartments, with the most prominent shortening found at the +4 to +7 positions ( Fig. 3k ). These results are in line with recent findings showing telomere shortening associated with TRF1 deletion in the hematopoetic system as the result of increased compensatory proliferation of the remaining stem cell pools [5] . In support of this notion, we also found higher numbers of cells positive for phosphorylated histone 3, a marker for late S phase and mitosis, in the TRF1 lox/lox intestinal crypts compared with the controls ( Supplementary Fig. S7c ). High TRF1 levels are associated with pluripotency To address TRF1 regulation in pluripotent cells, we first generated iPS cells from MEFs of the different genotypes, which were able to give rise to chimeric mice upon morulae aggregation ( Supplementary Fig. S8a and Supplementary Table S1 ), demonstrating that they were indeed pluripotent. Similar to MEFs, the eGFP–TRF1 fusion protein was located at telomeres in iPS cells as indicated by chromatin immunoprecipitation (ChIP) ( Supplementary Fig. S9a,b ; Methods). As expected, eGFP–TRF1 abundance at telomeres was half in heterozygous eGFP–TRF1 +/KI cells compared with eGFP–TRF1 KI/KI cells ( Supplementary Fig. S9a,b ). Furthermore, expression of the eGFP–TRF1 fusion protein did not interfere with endogeneous TRF1 expression in iPS cells, as indicated by western blot analysis ( Supplementary Fig. S9c ). Finally, mass spectroscopy of protein complexes immunoprecipitated with an anti-GFP antibody in eGFP–TRF1 KI/KI , eGFP–TRF1 +/KI and eGFP–TRF1 +/+ iPS cells showed co-immunoprecipitation of the different components of shelterin, namely TPP1, RAP1, TRF1, TIN2 and POT1 (ref. 2 ) in eGFP–TRF1 KI/ and eGFP–TRF1 +/KI iPS cells ( Supplementary Fig. S9d ), thus demonstrating that the eGFP–TRF1 fusion protein interacts with telomeric repeats and with other members of the shelterin complex in iPS cells. Next, we studied regulation of endogenous TRF1 as well as of the eGFP–TRF1 fusion protein in iPS cells compared with the parental MEFs. We found that the endogenous TRF1 protein was highly increased in wild-type iPS cells compared with the parental MEFs, as indicated by western blotting analysis ( Fig. 4a ). Indeed, the increase of TRF1 expression was in the same range to that of the pluripotency genes Oct3/4 and Nanog ( Fig. 4a ). Endogenous TRF1 was also increased in heterozygous eGFP–TRF1 +/KI iPS, although to lower levels than eGFP–TRF1 KI/KI iPS cells owing to the presence of a single copy of the endogenous TRF1 gene, and was undetectable in homozygous eGFP–TRF1 KI/KI iPS cells ( Fig. 4a ). Inversely, the eGFP–TRF1 protein was upregulated to the highest levels in eGFP–TRF1 KI/KI iPS cells, to half the levels in heterozygous eGFP–TRF1 +/KI iPS, and was undetectable in wild-type iPS cells ( Fig. 4a ). These findings were confirmed by fluorescence-activated cell sorting (FACS) analysis, which showed that the eGFP intensity in eGFP–TRF1 KI/KI was approximately double than that of eGFP–TRF1 +/KI ( Fig. 4c ). FACS analysis also confirmed similarly high Nanog expression in iPS cells of the three genotypes ( Fig. 4d ), supporting that the different genotype iPS cells were indeed pluripotent. 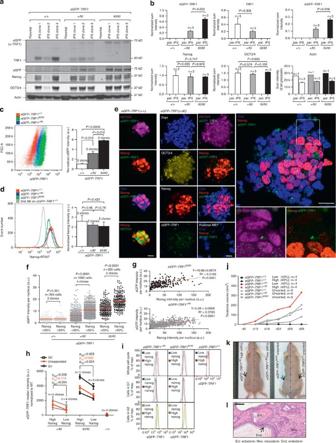Figure 4: TRF1 expression increases during reprogramming and correlates with pluripotency. (a,b) Western blotting against eGFP, TRF1, Nanog, OCT3/4 and actin of nuclear fractions of passage 3 parental MEFs (par.) and independent iPS clones (passage 5).n, independent clones. Error bars: s.e.m. Statistical analysis: two-sided Student’st-test. (c,d) FACS analysis of iPS cells (passage 7) confirming the eGFP-TRF1 (c) and Nanog (d) expression levels shown inaandb. Error bars: s.e.m. Statistical analysis: two-sided Student’st-test. (e) IPS colonies (passage 6) stained with antibodies against Nanog and OCT3/4. Note, the eGFP–TRF1 expression pattern is similar to that of Nanog. IPS passage number: 6. Scale bars, 25 μm. (f,g) Positive correlations between eGFP–TRF1 fluorescence intensity and Nanog expression levels ineGFP–TRF1+/KIandeGFP–TRF1KI/KIiPS cells (passage 6). Analysis of mean eGFP–TRF1 and Nanog fluorescence per nucleus. Statistical comparison: two-sided Student’st-test (f). Linear regression analysis (g). (h,i) FACS analysis of wild-type,eGFP–TRF1+/KIandeGFP–TRF1KI/KIiPS cells (passage 7) grouped into Nanoglow- and Nanoghigh-expressing cells (1:1) depending on the cell-cycle phase. A positive correlation between eGFP–TRF1 expression and Nanog expression is found, similar tofandg. Error bars: s.e.m. Statistical analysis: one-sided (known tendency) Student’st-test. (j) Teratoma formation by iPS cells (passage 4) unsorted (grey) and sorted for high and low eGFP–TRF1 expression in G1 phase of the cell cycle (red). From the sorted cells, onlyeGFP–TRF1+/KIhigh iPS cells formed teratomas. Of the unsorted cells, all the genotypes formed teratomas with a later onset and smaller volumes. The earlier teratoma onset of the sorted eGFP–TRF1highiPS cells indicates that high eGFP–TRF1 expression marks a subpopulation of more undifferentiated cells within the bulk iPS cells. Mean tumour volumes per genotype and days after injection are depicted.n, flanks injected. (k) Representative images of mice injected with unsorted wild-type andeGFP–TRF1KI/KIiPS cells (top picture) and sorted high and loweGFP–TRF+/KIiPS cells (bottom). (l) Representative image of aneGFP–TRF1+/KIteratoma stained for haematoxylin and eosin showing all three germ layers (endoderm: end; mesoderm: mes; ectoderm: ect). Scale bar, 100 μm. Figure 4: TRF1 expression increases during reprogramming and correlates with pluripotency. ( a , b ) Western blotting against eGFP, TRF1, Nanog, OCT3/4 and actin of nuclear fractions of passage 3 parental MEFs (par.) and independent iPS clones (passage 5). n , independent clones. Error bars: s.e.m. Statistical analysis: two-sided Student’s t- test. ( c , d ) FACS analysis of iPS cells (passage 7) confirming the eGFP-TRF1 ( c ) and Nanog ( d ) expression levels shown in a and b . Error bars: s.e.m. Statistical analysis: two-sided Student’s t- test. ( e ) IPS colonies (passage 6) stained with antibodies against Nanog and OCT3/4. Note, the eGFP–TRF1 expression pattern is similar to that of Nanog. IPS passage number: 6. Scale bars, 25 μm. ( f , g ) Positive correlations between eGFP–TRF1 fluorescence intensity and Nanog expression levels in eGFP–TRF1 +/KI and eGFP–TRF1 KI/KI iPS cells (passage 6). Analysis of mean eGFP–TRF1 and Nanog fluorescence per nucleus. Statistical comparison: two-sided Student’s t- test ( f ). Linear regression analysis ( g ). ( h , i ) FACS analysis of wild-type, eGFP–TRF1 +/KI and eGFP–TRF1 KI/KI iPS cells (passage 7) grouped into Nanog low - and Nanog high -expressing cells (1:1) depending on the cell-cycle phase. A positive correlation between eGFP–TRF1 expression and Nanog expression is found, similar to f and g . Error bars: s.e.m. Statistical analysis: one-sided (known tendency) Student’s t- test. ( j ) Teratoma formation by iPS cells (passage 4) unsorted (grey) and sorted for high and low eGFP–TRF1 expression in G1 phase of the cell cycle (red). From the sorted cells, only eGFP–TRF1 +/KI high iPS cells formed teratomas. Of the unsorted cells, all the genotypes formed teratomas with a later onset and smaller volumes. The earlier teratoma onset of the sorted eGFP–TRF1 high iPS cells indicates that high eGFP–TRF1 expression marks a subpopulation of more undifferentiated cells within the bulk iPS cells. Mean tumour volumes per genotype and days after injection are depicted. n , flanks injected. ( k ) Representative images of mice injected with unsorted wild-type and eGFP–TRF1 KI/KI iPS cells (top picture) and sorted high and low eGFP–TRF +/KI iPS cells (bottom). ( l ) Representative image of an eGFP–TRF1 +/KI teratoma stained for haematoxylin and eosin showing all three germ layers (endoderm: end; mesoderm: mes; ectoderm: ect). Scale bar, 100 μm. Full size image In summary, both the endogenous TRF1 locus and the KI eGFP–TRF1 locus are dramatically activated upon induction of pluripotency, in a fashion that resembles that of the Oct3/4 and Nanog pluripotency genes. Of note, the increased TRF1 levels associated with pluripotency were not paralleled to the same extent by other shelterin proteins, such as TRF2 or RAP1 ( Supplementary Fig. S10a,b ). TRF1 correlates with Nanog in iPS cells Next, we studied the distribution of eGFP fluorescence in different genotype iPS cell clones compared with parental MEFs. In agreement with the western blot results, average eGFP–TRF1 fluorescence per nucleus was increased in eGFP–TRF1 +/KI and eGFP–TRF1 KI/KI iPS colonies compared with the parental MEFs ( Supplementary Fig. S11a,b ). Again, EGFP–TRF1 KI/KI iPS colonies showed approximately double the amount of eGFP than the eGFP–TRF1 +/KI iPS colonies ( Supplementary Fig. S11b ). We also observed a significant increase in telomere length in all genotypes, in agreement with telomere elongation during reprogramming ( Supplementary Fig. S11c ) [9] . Intriguingly, eGFP–TRF1 fluorescence greatly varied in different cells of the same iPS cell colony ( Fig. 4e ). To understand the nature of this cell-to-cell eGFP–TRF1 heterogeneity within iPS cell colonies, we performed double immunofluorescence with eGFP and Nanog antibodies. It has been previously reported that Nanog levels fluctuate and are not homogenous within ES and iPS cell cultures [33] , [34] . Interestingly, we observed a positive correlation between Nanog and eGFP–TRF1 protein levels in eGFP–TRF1 +/KI and eGFP–TRF1 KI/KI nuclei ( Fig. 4e–g ). In addition, iPS cells showing >50% higher eGFP–TRF1 expression also showed more Nanog expression than those with <50% eGFP fluorescence ( Fig. 4f ). We confirmed this positive correlation between Nanog and eGFP–TRF1 by using flow cytometry analysis ( Fig. 4h ). In particular, we separated the eGFP–TRF1-expressing cells into high and low Nanog-expressing cells (ratio 1:1), and found increased eGFP–TRF1 expression in the Nanog high compared with Nanog low cells both in heterozygous-KI and homozygous-KI iPS cells ( Fig. 4h ). Of note, a similar correlation was not observed in the case of Oct3/4 protein levels, which are also greatly upregulated in iPS colonies ( Fig. 4e ). Next, we addressed whether the positive correlation between eGFP–TRF1 and Nanog occurred at the transcriptional level. To this end, we sorted iPS cells into high and low eGFP–TRF1-expressing cells (1:1) and analysed Nanog messenger RNA levels by quantitative real-time reverse transcriptase PCR (RT–qPCR). First, we confirmed increased eGFP–TRF1 mRNA levels in heterozygous-KI and homozygous-KI iPS cells compared with wild-type iPS cells, with eGFP–TRF1 +/KI iPS cells showing approximately half the expression than eGFP–TRF1 KI/KI iPS cells ( Supplementary Fig. S12a ). Interestingly, eGFP high iPS cells showed more mRNA Nanog expression than eGFP low cells in both heterozygous-KI and homozygous-KI clones ( Supplementary Fig. S12a ). As control, Nanog mRNA was undetectable in wild-type MEFs and greatly elevated in the corresponding wild-type iPS cells ( Supplementary Fig. S12a ). Of note, Oct3/4 mRNA levels were similar in eGFP high iPS cells and eGFP low iPS cells in both heterozygous-KI and homozygous-KI clones. Interestingly, eGFP–TRF1 low iPS cells that were grown for 3 days in gelatin-coated dishes were capable of re-establishing new iPS cell colonies with high expression of Nanog and of eGFP–TRF1 ( Supplementary Fig. S12b ), suggesting that high TRF1 levels can be re-established. This behaviour is similar to that observed for cells with low amounts of Nanog, which can give rise to iPS cell colonies with heterogeneous Nanog levels again [34] . Also in agreement with eGFP–TRF1 high marking pluripotent cells within iPS populations, we found elevated TERT mRNA levels in eGFP high iPS cells compared with eGFP low iPS cells [35] . Elevated TERT expression in the eGFP high iPS cells also correlated with longer telomeres in these cells compared with the eGFP low iPS cells ( Supplementary Fig. S12c ). In summary, both the pluripotency marker Nanog and TERT levels and telomere length are increased in the eGFP high iPS cells compared with eGFP low iPS cells, suggesting that elevated eGFP–TRF1 mRNA levels correlate with increased pluripotency. Finally, we addressed whether the higher amounts of eGFP–TRF1 in pluripotent iPS cells were associated with the pluripotent state per se or could be related to increased division rates in these cells. To this end, we grew iPS cells on gelatin-coated dishes in a medium containing fetal bovine serum (FBS), which is known to induce increased proliferation and loss of pluripotency [36] , [37] . As expected, iPS cells grown under these conditions showed increased proliferation rates ( Supplementary Fig. S13a ). Interestingly, eGFP–TRF1 expression was decreased in both eGFP–TRF1 +/KI and eGFP–TRF1 KI/KI iPS cells after 4 days in FBS ( Supplementary Fig. S13a,b ), concomitant with a change in cell morphology towards a more differentiated state ( Supplementary Fig. S13c ) and decreased expression of the Nanog and Oct3/4 pluripotency factors in eGFP–TRF1 +/KI iPS cells ( Supplementary Fig. S13d,e ). These findings indicate that high eGFP–TRF1 expression in iPS cells is associated with pluripotency rather than to high proliferation rates. eGFP–TRF1 high iPS cells have higher pluripotency potential To further determine the properties of eGFP high iPS cells compared with eGFP low iPS cells, we tested their respective abilities to form chimeras and teratomas, an indication of their pluripotency potential. To this end, we sorted eGFP high and eGFP low iPS cells in the same phase of the cell cycle (G1 state cells) and with the same DNA content from eGFP–TRF1 +/KI iPS cell populations, in this manner avoiding possible differences in telomere numbers and therefore TRF1 levels. For teratoma formation, we injected the 40% of iPS cells with the highest and lowest eGFP–TRF1 fluorescence after sorting into the flanks of nude mice. Strikingly, only the eGFP–TRF1 high -sorted iPS cells were capable of forming teratomas and no teratomas were obtained with the eGFP–TRF1 low -sorted iPS ( Fig. 4j ). Furthermore, teratomas obtained from eGFP–TRF1 high -sorted iPS cells showed all three germ layers indicating that they are pluripotent ( Fig. 4l ). Interestingly, we observed that expression of eGFP–TRF1 highly correlated with the expression of Nanog in teratoma sections, so that the undifferentiated areas expressed higher amounts of eGFP–TRF1 compared with more differentiated areas ( Supplementary Fig. S14a–c ), suggesting that TRF1 expression is an indicator of the degree of differentiation within the tumour. A similar finding was made when we aggregated morulae with iPS cells with either high eGFP–TRF1 content or low eGFP–TRF1 content. EGFP–TRF1 high iPS cells were able to give rise to chimeric mice with high chimerism whereas iPS cells with low or undetectable amounts of eGFP–TRF1 were not potent enough to give rise to chimeric mice ( Supplementary Fig. S15 and Supplementary Table S2 ). Together, these results support the notion that TRF1 expression levels are indicative of the level of pluripotency of iPS cells. Thus, the higher the expression levels of TRF1, the higher the pluripotency potential. eGFP–TRF1 levels do not correlate with telomere length Previous work from our laboratory showed that during the generation of iPS cells, telomeres undergo a net telomere elongation that continues post reprogramming until reaching the hyper-long telomeres of ES cells [9] . Here, we took advantage of this phenomenon to address whether eGFP–TRF1 fluorescence correlated with telomere length in vivo . To this end, we first determined telomere length at different passage iPS cells by using telomere quantitative fluorescence in situ hybridization (Q-FISH) directly on fixed iPS colonies (Methods). iPS cells (P7) from all the three genotypes were able to elongate telomeres to a similar extend than the corresponding parental MEFs ( Supplementary Fig. S16a–c ). Strikingly, however, while wild-type and eGFP–TRF1 +/KI telomeres continued growing with increasing passages until reaching hyper-long ES cell telomeres at passage 36, the telomeres of eGFP–TRF1 homozygous iPS cells ceased to further elongate between passage 7 and 16 ( Supplementary Fig. S16c ). The inability of eGFP–TRF1 KI/KI iPS cell telomeres to show further elongation might be related to inadequate telomere replication and increased telomere fragility (MTS) in this genotype, or, alternatively, may suggest a role of TRF1 in telomerase recruitment, which is partially impaired in the eGFP–TRF1 fusion protein. In this regard, TPP1, a TRF1-interacting protein, was previously described by us to be required for telomerase-mediated telomere elongation during reprogramming [10] . In summary, these results highlight the importance of TRF1 for telomere length maintenance in vivo [38] , [39] . Next, we measured eGFP–TRF1 intensity per telomere and per nucleus to address whether it was directly correlated with telomere length changes during reprogramming. However, a linear correlation between telomere length and eGFP intensity was not observed. In particular, while telomere length increased by about 1.7-fold when comparing MEFs with iPS cells at passage 7 ( Supplementary Fig. S16b ), the eGFP intensity increased by 20-fold at this point ( Supplementary Fig. S17a,b ). Furthermore, while eGFP–TRF1 levels were maintained stable from passage 7 onwards, the telomeres of WT and heterozygous cells kept elongating until passage 36 ( Supplementary Figs S16b,c and S17b,c ). This suggests that increased TRF1 at the induction of pluripotency precedes telomere elongation, again in line with the notion that elevated TRF1 levels are characteristic of the pluripotent state and uncoupled from telomere elongation. TRF1 is essential for reprogramming To further address whether TRF1 levels are uncoupled from telomerase-dependent telomere elongation during reprogramming, we studied TRF1 protein levels during reprogramming of MEFs deficient for Tpp1 ( Tpp1 Δ/Δ Cre-shp53 ), previously shown by us to show impaired telomere elongation in iPS cells [10] . Strikingly, TRF1 levels were highly upregulated in Tpp1 Δ/Δ Cre-shp53 iPS cells compared with the parental MEFs, reaching similarly high levels than those of wild-type controls even though the resulting iPS cells failed to elongate their telomeres ( Fig. 5a ) [10] . These results clearly demonstrate that TRF1 upregulation at the induction of pluripotency is uncoupled from telomere elongation. 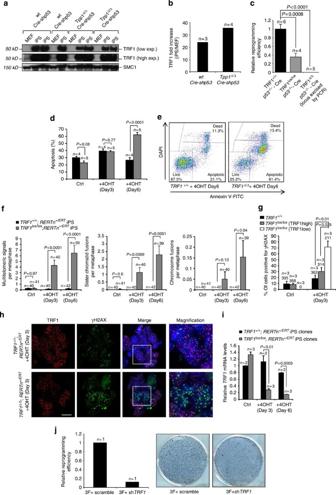Figure 5: High TRF1 levels during reprogramming are essential for the generation of iPS cell clones. (a,b) TRF1 is highly overexpressed in iPS cells, even in the absence of telomere elongation. (a) Expression of TRF1 in wild-type andTpp1Δ/ΔMEF and iPS cells as detected by western blot. Note that TRF1 expression is highly increased in iPS cells if compared with parental MEF, even inTpp1Δ/ΔiPS cells that do not elongate telomeres during reprogramming. SMC1 was used as a loading control for nuclear extract. (b) Quantification of TRF1 ofa, relative to SMC1.n, independent iPS clones. (c) Relative reprogramming efficiencies of the indicated cells. Note that the only iPS colonies obtained from theTRF1lox/lox-Cre MEFs came from cells withoutTRF1excision.n, independent experiments. Error bars: s.e.m. Statistical analysis: two-sided Student’st-test. (d) Apoptosis was determined on control-treated iPS cells and iPS cells at day 3 and 6 of 4-OHT treatment.n, iPS clones analysed. Error bars: s.e.m. Statistical analysis: two-sided Student’st-test. (e) Representative FACS profiles at day 6 of 4-OHT treatment. (f) Frequency of aberrations in metaphase spreads of the indicated genotypes and conditions.n, metaphases from a total of two iPS clones per genotype. Error bars: s.e.m. Statistical analysis: two-sided Student’st-test. (g) Percentage of γH2AX-positive cells in non-treated (Ctrl) and 4-OHT-treated (Day 3) iPS cells.n, iPS clones used for the analysis. The total number of cells analysed per genotype is shown. Error bars: s.e.m. Statistical analysis: two-sided Student’st-test. (h) Representative images of TRF1 and γH2AX immunofluorescence co-staining. Scale bar, 10 μm. (i) mRNA levels ofTRF1decrease with time of 4-OHT treatment at day 3 and day 6. Ctrl are control-treated cells at day 3 where no difference in theTRF1mRNA levels was detected. Error bars: s.e.m. Statistical analysis: two-sided Student’st-test. (j) Left panel: relative reprogramming efficiency of the indicated cells. Note that shRNA-TRF1-transduced MEF show decreased reprogramming capacity.n, number of independent MEF. Right panel: reprogramming plates stained with alkaline phosphatase. Figure 5: High TRF1 levels during reprogramming are essential for the generation of iPS cell clones. ( a , b ) TRF1 is highly overexpressed in iPS cells, even in the absence of telomere elongation. ( a ) Expression of TRF1 in wild-type and Tpp1 Δ/Δ MEF and iPS cells as detected by western blot. Note that TRF1 expression is highly increased in iPS cells if compared with parental MEF, even in Tpp1 Δ/Δ iPS cells that do not elongate telomeres during reprogramming. SMC1 was used as a loading control for nuclear extract. ( b ) Quantification of TRF1 of a , relative to SMC1. n , independent iPS clones. ( c ) Relative reprogramming efficiencies of the indicated cells. Note that the only iPS colonies obtained from the TRF1 lox/lox -Cre MEFs came from cells without TRF1 excision. n , independent experiments. Error bars: s.e.m. Statistical analysis: two-sided Student’s t- test. ( d ) Apoptosis was determined on control-treated iPS cells and iPS cells at day 3 and 6 of 4-OHT treatment. n , iPS clones analysed. Error bars: s.e.m. Statistical analysis: two-sided Student’s t- test. ( e ) Representative FACS profiles at day 6 of 4-OHT treatment. ( f ) Frequency of aberrations in metaphase spreads of the indicated genotypes and conditions. n , metaphases from a total of two iPS clones per genotype. Error bars: s.e.m. Statistical analysis: two-sided Student’s t- test. ( g ) Percentage of γH2AX-positive cells in non-treated (Ctrl) and 4-OHT-treated (Day 3) iPS cells. n , iPS clones used for the analysis. The total number of cells analysed per genotype is shown. Error bars: s.e.m. Statistical analysis: two-sided Student’s t- test. ( h ) Representative images of TRF1 and γH2AX immunofluorescence co-staining. Scale bar, 10 μm. ( i ) mRNA levels of TRF1 decrease with time of 4-OHT treatment at day 3 and day 6. Ctrl are control-treated cells at day 3 where no difference in the TRF1 mRNA levels was detected. Error bars: s.e.m. Statistical analysis: two-sided Student’s t- test. ( j ) Left panel: relative reprogramming efficiency of the indicated cells. Note that shRNA-TRF1-transduced MEF show decreased reprogramming capacity. n , number of independent MEF. Right panel: reprogramming plates stained with alkaline phosphatase. Full size image Next, we set to determine whether TRF1 itself showed the behaviour of a pluripotency gene and was essential for the reprogramming of MEFs into iPS cells. To this end, we reprogrammed MEFs deficient for TRF1 and simultaneously abrogated for p53, TRF1 Δ/Δ p53 −/− -Cre MEFs, which we previously demonstrated to rescue proliferative defects associated with TRF1 deficiency in vivo as well as to facilitate the reprogramming of cells with severe telomeric damage [6] , [8] . Strikingly, we repeatedly failed to obtain any iPS cell colonies in the TRF1 Δ/Δ p53 −/− -Cre cultures ( Fig. 5c ), and the few colonies obtained in the case of TRF1 lox/lox p53 −/− -Cre cultures came from cells without TRF1 excision ( Fig. 5c and Supplementary Fig. S18a ), indicating that TRF1 deficiency completely blocks reprogramming, even in the absence of p53. In line with this, TRF1 deficiency prevented some of the key events associated with reprogramming, such as appearance of SSEA-1-expressing clones ( Supplementary Fig. S18b ) [40] and high expression of the pluripotency genes Nanog and Oct3/4 at the time of appearance of the first iPS clones 14 days post infection ( Supplementary Fig. S18c ). Given the essential role of TRF1 for reprogramming, we sought to determine whether TRF1 was capable to regulate gene expression of crucial pluripotency genes. In this regard, the shelterin Rap1 has been described to bind extra-telomeric sites along the genome and to regulate gene expression [41] . To this end, we performed TRF1 ChIP-sequencing analysis in both MEFs and iPS cells. As expected for TRF1-binding telomeres, we found a robust enrichment in telomere tracts, which was greater in cells with longer telomeres ( Supplementary Fig. S19a ; compare passage 5 and 30 iPS cells and MEF versus iPS). Despite having a good read distribution along peaks ( Supplementary Fig. S19b ), we did not find any significant TRF1 binding to putative regulatory regions nor intragenic binding of TRF1 outside telomeric regions ( Supplementary Tables S3–S5 ). These results indicate that TRF1 does not influence reprogramming through a direct role in transcriptional regulation. Chromosomal instability in TRF1-deficient iPS cells Next, we wondered whether TRF1 could be essential not only during the acquisition of pluripotency but also during the maintenance of the pluripotent state. To this end, we generated TRF1 -null iPS cells using primary MEFs carrying a conditional loxP-flanked TRF1 allele and an inducible Cre-ERT2 recombinase allele ( RERTn). After reprogramming of TRF1 lox/lox ;RERTn +/ERT and TRF1 +/+ ;RERTn +/ERT MEFs, the resultant iPS cells were replated in the presence of 4-hydroxytamoxifen (4-OHT) to obtain TRF1ko and TRF1wt iPS cells, respectively. It has been previously described that TRF1 deficiency in MEFs induces telomere uncapping, telomere fragility (MTS) and a rapid induction of cell-cycle arrest and senescence, mediated by the p53 and pRb pathways activation [6] . As iPS cells are very sensitive to DNA damage, we checked whether TRF1ko iPS cells undergo apoptosis. At day 3 and 6 of 4-OHT treatment, we observed an increase in apoptosis in TRF1 Δ/Δ ; RERTn +/ERTOHT iPS cells compared with the TRF1 +/+ ; RERTn +/ERTOHT iPS cells, while there was no significant differences in control-treated iPS cells ( Fig. 5d ). To address whether TRF1 deficiency causes telomeric aberrations in iPS cells, we performed telomeric Q-FISH on metaphases (Methods). As expected, TRF1 Δ/Δ ; RERTn +/ERTOHT iPS cells showed higher levels of MTS, sister-chromatid and chromosome fusions at day 3 and day 6 after 4-OHT treatment ( Fig. 5f ), suggesting increased telomere fragility and telomere uncapping, respectively, due to TRF1 abrogation. Next, we analysed DDR activation by co-staining of γH2AX and TRF1 in iPS cells at day 3 of 4-OHT treatment. We detected a considerable increase in the percentage of γH2AX-positive cells ( Fig. 5g ) in TRF1 Δ/Δ ; RERTn +/ERTOHT with low levels of TRF1 compared with TRF1 +/+ ; RERTn +/ERTOHT and TRF1 Δ/Δ ; RERTn +/ERTOHT with high levels of TRF1, in agreement with the results from TRF1 -null MEFs. Finally, we confirmed TRF1 abrogation in TRF1 Δ/Δ ; RERTn +/ERTOHT iPS cells by qRT–PCR ( Fig. 5i ) at day 3 and 6 of 4-OHT treatment. In view that TRF1 deficiency completely blocks reprogramming, even in the absence of p53 ( Fig. 5c ), we set to confirm this essential role for TRF1 in reprogramming by knocking down TRF1 expression during the reprogramming process. To this end, p53 −/− MEFs were reprogrammed using a cocktail of retroviral vectors expressing the three reprogramming factors (Oct3/4, Klf4 and Sox2) and a lentiviral vector expressing either TRF1 short-hairpin RNA (shRNA) or a scramble shRNA as a control. Our results indicate that a reduced expression of TRF1 during reprogramming strongly decreases the reprogramming capacity of the cells ( Fig. 5j ). In line with this, we found an increased intensity of γH2AX per nucleus in cells with reduced levels of TRF1 ( Supplementary Fig. S20a ), suggesting that increased DNA damage may be responsible for the deficient reprogramming capacity of these cells. Similarly, we observed a significant increase in MTS at day 17 post infection, but not at an earlier time point (day 10 post infection), in cells deficient for TRF1 when compared with cells with normal levels of TRF1 ( Supplementary Fig. S20b ), suggesting that accumulation of MTS may be associated with the number of cell doublings to form an iPS cell colony. Together, these findings indicate that TRF1 is essential both for the induction and maintenance of pluripotency in iPS cells. Oct3/4 modulates TRF1 expression Next, we set to address the mechanism by which TRF1 is upregulated upon the induction of pluripotency. First, we followed TRF1 expression during reprogramming of wild-type MEFs by using qRT–PCR. TRF1 mRNA levels were increased as early as 3 days after addition of the reprogramming cocktail to MEFs ( Supplementary Fig. S21a ). In contrast, Nanog mRNA levels started to significantly increase only after 6–9 days of reprogramming ( Supplementary Fig. S20b ), arguing that TRF1 is not a target of Nanog. Instead, recent ChIP-sequencing experiments in mouse ES cells (mESC) showed that the pluripotency factor Oct3/4 can bind to TRF1 promoter regions [42] , suggesting that Oct3/4 could be responsible for TRF1 upregulation during reprogramming. To directly test this, we transduced wild-type MEFs with each of the reprogramming factors (Oct3/4, Sox2 and Klf4) (see Methods). Interestingly, 3 days after infection, we detected a significant increase in TRF1 levels in Oct3/4-transduced MEFs only, even in the absence of reprogramming ( Fig. 6a ). Of note, even though Oct3/4 was sufficient to induce TRF1 in MEFs, TRF1 levels in established iPS were still significantly higher ( Fig. 6a ). These results suggest that Oct3/4 is sufficient to induce TRF1 upregulation during the reprogramming process, but additional factors may be required for full TRF1 induction in iPS cells. 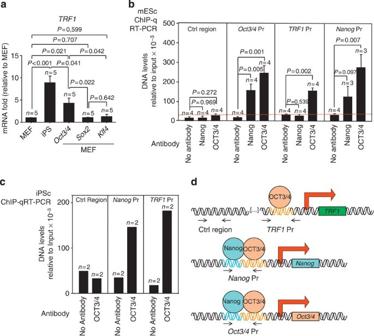Figure 6: OCT3/4 modulates TRF1 expression in pluripotent cells by directly binding toTRF1promoter. (a)TRF1transcription levels in MEFs transduced with eitherOct3/4,Sox2orKlf4, as estimated by qRT–PCR. The mRNA fold increase relative toTRF1levels in wild-type MEFs 3 days after transduction with the indicated retroviral vectors is depicted. Note thatOct3/4is the only factor able to increase TRF1 levels in the absence of cellular reprogramming. Non-transduced MEFs and wild-type iPS cells are included for reference.n, independent MEF clones used per condition. Error bars: s.e.m. Statistical analysis: two-sided. Student’st-test. (b,c) DNA levels, as measured by qRT–PCR after ChIP in mESc (b) or iPSc (c). The amount of DNA in each ChIP was normalized to its corresponding input DNA levels (total genomic DNA not subjected to immunoprecipitation). The antibodies used are indicated under each bar. The regions amplified by qRT–PCR are indicated on top of the panels (Ctrl Region, control region;Oct3/4-Pr,Oct3/4promoter;TRF1-Pr,TRF1promoter; andNanog-Pr,Nanogpromoter). Note that OCT3/4 binds toTRF1,NanogandOct3/4promoters, while Nanog does only bind toNanogandOct3/4promoters but not that ofTRF1.n, independent immunoprecipitations performed. Error bars: s.e.m. Statistical analysis: two-sided. Student’st-test. (d) Schematic representation of the genomic regions and primer pairs used for the ChIP–qRT–PCR analysis described inbandc. Figure 6: OCT3/4 modulates TRF1 expression in pluripotent cells by directly binding to TRF1 promoter. ( a ) TRF1 transcription levels in MEFs transduced with either Oct3/4 , Sox2 or Klf4 , as estimated by qRT–PCR. The mRNA fold increase relative to TRF1 levels in wild-type MEFs 3 days after transduction with the indicated retroviral vectors is depicted. Note that Oct3/4 is the only factor able to increase TRF1 levels in the absence of cellular reprogramming. Non-transduced MEFs and wild-type iPS cells are included for reference. n , independent MEF clones used per condition. Error bars: s.e.m. Statistical analysis: two-sided. Student’s t- test. ( b , c ) DNA levels, as measured by qRT–PCR after ChIP in mESc ( b ) or iPSc ( c ). The amount of DNA in each ChIP was normalized to its corresponding input DNA levels (total genomic DNA not subjected to immunoprecipitation). The antibodies used are indicated under each bar. The regions amplified by qRT–PCR are indicated on top of the panels (Ctrl Region, control region; Oct3/4 -Pr, Oct3/4 promoter; TRF1 -Pr, TRF1 promoter; and Nanog -Pr, Nanog promoter). Note that OCT3/4 binds to TRF1 , Nanog and Oct3/4 promoters, while Nanog does only bind to Nanog and Oct3/4 promoters but not that of TRF1 . n , independent immunoprecipitations performed. Error bars: s.e.m. Statistical analysis: two-sided. Student’s t- test. ( d ) Schematic representation of the genomic regions and primer pairs used for the ChIP–qRT–PCR analysis described in b and c . Full size image Interestingly, while putative Nanog and Oct3/4-binding sites have been found at the human TRF1 promoter, mouse cells only show a putative Oct3/4-binding site ( Supplementary Fig. S21c ; Source ENSEMBL (ref. 42 )). Thus, we set to address whether Oct3/4 and/or Nanog were able to directly bind to the mouse TRF1 promoter in pluripotent cells. To this end, we performed ChIP–qRT–PCR experiments in mES cells and iPSc ( Fig. 6b–d ). In particular, we immunoprecipitated Oct3/4- and Nanog-bound chromatin and detected either Oct3/4 promoter (Oct3/4-Pr), Nanog promoter (Nanog-Pr), TRF1 promoter (TRF1-Pr) or an unrelated control region upstream of the TRF1 promoter (Ctrl region) ( Fig. 6d ). In mESc, we detected significant binding of Oct3/4 protein to Oct3/4-Pr, Nanog-Pr and TRF1-Pr. We also detected Nanog binding to its own promoter and that of Oct3/4, but failed to detect Nanog binding to the TRF1-Pr ( Fig. 6b ). We confirmed these results in iPS cells ( Fig. 6c ). Together, these results demonstrate that Oct3/4 can directly regulate TRF1 levels together with bona fide pluripotency markers such as Nanog or Sox2 in an orchestrated manner, supporting the hypothesis that TRF1 is an essential protein during the acquisition of pluripotency. Here, we generated the first KI reporter mouse for a key component of the mammalian telomere protection complex, TRF1, the eGFP–TRF1 mouse model. Telomeres from cells and mice carrying the eGFP–TRF1 KI allele can be detected and followed in vivo by direct eGFP fluorescence. Here, we used this feature to understand the regulation and function of TRF1 in adult stem cell compartments as well as in pluripotent stem cells. The TRF1 reporter mouse is also likely to be instrumental for the study of the regulation of TRF1 in normal and pathological conditions (that is, cancer and aging), for identification of new TRF1 partners, as well as for tracking telomeres in living cells in response to different agents and stimuli. In particular, in the case of adult stem cell compartments, we find that eGFP–TRF1 expression is very high at the known stem cells compartments of the skin and the small intestine, and markedly decreased in the more differentiated compartments. Interestingly, we find that eGFP–TRF1 expression at the stem Lgr5-expressing cells of the small intestine crypt is uncoupled from telomere length, so that TRF1 levels but not telomere length is able to distinguish between the more primitive Lgr5+ cells and the more differentiated Lgr5− cells. Furthermore, we demonstrate that high TRF1 expression is not only a marker for the small intestine stem cell compartment but it is also essential for maintenance of tissue homeostasis. In particular, conditional TRF1 deletion in the small intestine leads to a rapid collapse of the intestinal villi/crypt structure, which is coincidental with increased DNA damage and apoptosis at the stem cell regions. Of note, the finding that cells with high TRF1 expression are enriched at two of the best characterized mouse adult stem cell compartments (skin and small intestine) suggest that eGFP–TRF1 reporter mice may represent a new tool for the isolation, identification and study of other adult stem cell populations in mice. In line with a role for TRF1 in stemness, we describe here that TRF1 is upregulated to similar levels than Nanog and Oct3/4 during the process of induction of pluripotency to generate iPS cells from parental MEFs. This is in agreement with a previous report showing that TRF1 is among of most upregulated genes associated with pluripotency [7] . Again, we show here that TRF1 induction during iPS cell generation is uncoupled from net telomere elongation, as indicated by induction of TRF1 in iPS cells defective for the shelterin component Tpp1 , previously shown by us to fail to elongate telomeres during reprogramming [10] . Importantly, we show here that high TRF1 levels are not only a property of pluripotent cells but also essential for reprogramming. In particular, TRF1-deficient MEFs completely fail to be reprogrammed, even in the absence of p53 (refs 6 , 8 ). Furthermore, conditional deletion of TRF1 in already established iPS cells leads to rapid elimination of iPS colonies coincidental with increased DNA damage and apoptosis, demonstrating that protection from telomere damage by TRF1 is essential for the maintenance of pluripotency. Together, these results suggest that TRF1 is an important factor for reprogramming of differentiated cells into iPS cells as well as for the maintenance of pluripotency. These results are in contrast to efficient reprogramming of cells with defective telomere elongation that owe to telomerase or Tpp1 deficiencies [8] , [10] , further suggesting that the essential role of TRF1 in reprogramming is unrelated to telomere maintenance. In summary, we describe here new roles for a telomere-protective protein, TRF1, in adult stem cells as well as pluripotent stem cells, which are independent of telomere length, and which highlight an essential role for telomere protection mediated by TRF1 in stem cell biology. On one hand, high TRF1 levels mark adult stem cell compartments as well as pluripotent stem cells. Moreover, TRF1 is essential both for maintenance of adult stem cell compartments of the small intestine and the skin, as well as for the induction and maintenance of pluripotency in iPS cells. Finally supporting the notion that TRF1 is a key factor for pluripotency, we make the unprecedented finding that TRF1 is a direct target of Oct3/4, which binds TRF1 promoter and is sufficient to upregulate TRF1, thus providing a mechanistic link between TRF1 and pluripotency. Generation of the eGFP–TRF1 KI mouse model The targeting construct and mice with the targeted TRF1 allele were generated by genOway (France). The neomycin-resistance (NEO) cassette was excised by crossing with mice carrying the Cre-recombinase. Mice of the wild-type, eGFP–TRF1 +/KI and eGFP–TRF1 KI/KI genotypes were generated and maintained at the CNIO mouse facility. The mice in this work are of mixed background: C57BL/6 (75%) and 129Sv (25%). All procedures performed on mice were revised and approved by the institutional Ethical Committee. Genotyping of the eGFP–TRF1 allele was performed by PCR as depicted with primers flanking the possible eGFP cassette. Forward primer: 5′-CAGGGTTAAATGCTCATGTTTATGGCG-3′; reverse primer: 5′-TGCTCTGGAGAATCCGAATCTGTCC-3′. Generation of MEFs and iPS cells Wild-type, eGFP–TRF1 +/KI and eGFP–TRF1 KI/KI : primary MEFs were isolated from E13.5 embryos. Generation of eGFP–TRF1 iPS cells from the indicated genotypes was performed as described [43] . The generation Tpp1 Δ/Δ iPS cells was described before [10] . TRF1 lox/lox ; p53 −/− and TRF1 +/+ ; p53 −/− MEFs were infected once with retroviral Cre-recombinase as described [6] . Puromycin (2 μg ml −1 ) selection was added 48 h after the infection. Selected cells were reprogrammed as described [8] . iPS colonies were picked 2–3 weeks after infection and expanded on feeder fibroblasts. Reprogramming and generation of TRF1-null iPS cells :. We reprogrammed TRF1 lox/lox and TRF1 +/+ ; RERTn +/ERT MEFs [44] as described above. The resulting iPS clones were picked and treated with with 4-OHT to obtain TRF1 Δ/Δ and TRF1 +/+ iPS cells, respectively. iPS from both genotypes were seeded at low density (50,000 cells per well in 6-well plates) in feeders or gelatin-coated (for qRT–PCR analysis) dishes, and treated with 4-OHT at a final concentration of 0.2 μM in complete iPS medium, which was replaced every day. TRF1 deletion in iPS obtained from TRF1 lox/lox p53 −/− Cre MEFs was checked by PCR with: forward primer: E1-popout 5′-ATAGTGATCAAAATGTGGTCCTGGG-3′; reverse primer: SA1 5′-GCTTGCCAAATTGGGTTGG-3′. Efficiency of reprogramming was determined by alkaline phosphatase activity (AP detection kit, Chemicon International), following the manufacturer’s instruction. Flow cytometry analysis Trypsinized iPS cells grown in knockout serum replacement (KSR)–ES–medium were washed in PBS supplemented with 1% FBS, fixed in 3% PFA at room temperature for 15 min and permeabilized with PBS +0.1% Triton-X100 followed by a PBS+1% FBS blocking step. Nanog expression was determined using an α-Nanog antibody at 1:200 dilution (Novus; NB100-58842) at room temperature for 45 min, followed by a secondary antibody labelled with AlexaF647. SSEA-1 expression during reprogramming was assessed by flow cytometry, as described [48] . Samples were acquired on a FACS Canto-II or a LSRII Fortessa (for SSEA-1) (BD, San Jose, CA) using pulse processing to exclude cell aggregates and debris. At least 20,000 events were collected per sample. Data were analysed using FlowJo Software v.9.1 (Treestar, Eugene, OR). FACS sorting For mRNA levels, IPS cells were trypsinized and washed in PBS with 1% FBS and re-suspended in DMEM 1 unit ml −1 LIF, 3% KSR and 3 mM EDTA. Wild-type, eGFP–TRF1 +/KI and eGFP–TRF1 KI/KI cells were FACS sorted on an Aria II (BD) according to their eGFP–TRF1 levels of expression into high and low fraction (1/1). Cell aggregates and dead cells were excluded by using pulse processing and 4′,6-diamidino-2-phenylindole. 1 × 10 6 cells for each fraction were collected, centrifuged, washed with PBS and prepared for the following experiments. For eGFP–TRF1 level-dependent teratoma and chimera formation, iPS cells were grown on feeders. Cells were further trypsinized and incubated with 10 μg ml −1 Hoechst at a concentration of 1 × 10 6 cells per ml were further sorted for G1 phase and eGFP–TRF1 abundance. Quantitative real-time PCR Total RNA from cells was extracted with Trizol (Life Technologies). Samples were treated with DNase I before reverse transcription, using random priming and iScript TM (BioRad) according to the manufacturer’s protocols (eGFP–TRF1 iPS cells) or using Ready-To-Go You-Prime First-Strand Beads kit (GE Healthcare). Quantitative real-time PCR was performed using an ABI PRISM 7700 (Applied Biosystems), using DNA Master SYBR-Green I mix (Applied Biosystems) according to the manufacturers protocol. All values were obtained in triplicates.Primers used are as follows:mNanog-F, 5′-AGGGTCTGCTACTGAGATGCTCTG-3′; mNanog-R, 5′-CAACCACTGGTTTTTCTGCCACCG-3′; mEndoOct3/4-R, 5′-TGCGGGCGGACATGGGGAGATCC-3′; mEndoOCT3/4-F, 5′-TCTTTCCACCAGGCCCCCGGCTC-3′; mTERT-F, 5′-GGATTGCCACTGGCTCCG-3′; mTERT-R, 5′-TGCCTGACCTCCTCTTGTGAC-3′; eGFP–TRF1-F, 5′-CCTGAGCAAAGACCCCAAC-3′; eGFP–TRF1-R, 5′-TCCTCCTGCTCTGGAGAATC-3′; m TRF1 -F: 5′-GTCTCTGTGCCGAGCCTTC-3′; m TRF1 -R: 5′-TCAATTGGTAAGCTGTAAGTCTGTG-3′; Gapdh-F, 5′-TTCACCACCATGGAGAAGGC-3′; Gapdh-R, 5′-CCCTTTTGGCTCCACCCT-3′; TRF1-Pr-F: 5′-GAAGGGGAAGAGGGAGTGAG-3′; TRF1-Pr-R: 5′-TTGTCAGGCACCTGTCTCAG-3′; TRF1-PrCtrlRegion-F: 5′-TCAGGAATGTCCCCTGAGAT-3′; TRF1-PrCtrlRegion-R: 5′-GCATTCCCTTCGGGTATTTT-3′; Nanog-Pr-F: 5′-GAAGGGGAAGAGGGAGTGAG-3′; Nanog-Pr-R: 5′-TTGTCAGGCACCTGTCTCAG-3′; OCT3/4-Pr-F: CTCTCGTCCTAGCCCTTCCT-3′; OCT3/4-Pr-R: 5′-CCTCCACTCTGTCATGCTCA-3′.Calculations were made using the ΔCt method as described in ref. 45 . Infection of MEFs for quantification of TRF1 mRNA levels Two days before infection, 4 × 10 5 293T cells were transfected with Fugene-6 (Roche) following manufacturer’s instructions and using 4 mg of pCL-Eco and 4 mg of each plasmid of interest (pMX-Sox2, pMX-KLF4 or pMX-OCT3/4). The day after, MEFs were seeded at a density of 2 × 10 5 cells in a p35 well and fresh media was added to the 293T cells. The following day, medium was collected, filtered through a 0,45 mm filter and 8 mg ml −1 polybrene was added; 1 ml of filtered medium was added to each well containing the MEFs seeded the day before; infection was repeated every 12 h to a total of four times and cells were harvested 3 days after the last infection for RNA isolation and subsequent qRT–PCR analysis. eGFP–TRF1 ChIP assay ChIP assays were performed as described [46] . In brief, after cross-linking and sonication, chromatin from 4 × 10 6 cells were used per immunoprecipitation with protein anti-GFP agarose beads (MBL International, D-153-8) and the following antibodies: 6 μg of anti-histone H3 (# ab1791, Abcam), 8 μl of polyclonal rabbit anti-TRF1 serum at (homemade and described in ref. 47 ). The immunoprecipitated DNA was transferred to a Hybond N+ membrane using a dot blot apparatus. The membrane was then hybridized with either a telomeric probe containing TTAGGG repeats or a probe recognizing major satellite sequences, which is characteristic of pericentric heterochromatin. Quantification of the signal was performed with ImageJ software (NIH). The amount of telomeric and pericentric DNA after ChIP was normalized for the total telomeric DNA. ChIP and quantitative real-time PCR ChIP and quantitative real-time PCR (ChIP–qPCR) was performed as previously described [41] . A total of 20 ng of total DNA were used in each qPCR reaction. SYBR-green reagent was used for qPCR following manufacturer’s instructions. Ct for every amplified region was normalized to its corresponding INPUT Ct, taking into account sample dilution for data representation. Antibodies used are as follows: Nanog 4 μg (Novus; NB100-58842); Oct3/4 (Santa Cruz sc-9081). Lentiviral transductions of the shRNAs Experiments were performed on MEFs from p53 −/− embryos (MEFs, of C57BL6 genetic background), reprogramming was performed as described above. For lentiviral transduction, retroviral supernatants were produced in HEK-293T cells (ATCC Number CRL-11268) (5 × 10 6 cells per 100-mm-diameter dish) transfected with the ecotropic packaging plasmid pCL-Eco (4 μg) together with either one of the following retroviral constructs (4 μg): pMXs-Klf4, pMXs-Sox2 or pMXs-Oct3/4 (obtained from Addgene) or pBabe Hygro (kindly donated by Francisco Real). Similarly, lentiviral supernatants were produced in HEK-293T cells (5 × 10 6 cells per 100-mm-diameter dish) transfected with the packaging plasmids pMDLg/pRRE (3.25 μg), pRSV.Rev (1.25 μg), pMD2.G VSVG (1.75 μg) (obtained from Addgene), and either one of the following shRNA lentiviral constructs (5 μg), pLKO.1-puro-scramble shRNA (obtained from Addgene) or pLKO.1-puro-TRF1 shRNA (bacterial glicerol stock (TRCM0000071298, obtained from Sigma-Aldrich). Transfections were performed using Fugene-6 transfection reagent (Roche) according to the manufacturer’s protocol. Two days later, viral supernatants (10 ml) were collected serially during the subsequent 48 h, at 12 h intervals, each time adding fresh medium to the cells (10 ml). The recipient MEFs had been seeded the previous day (2 × 105 cells per 60-mm-diameter dish) and received 1 ml of each of the corresponding viral supernatants. The following viral cocktails were used: pBabe Hygro and pLKO.1-puro-scramble shRNA (mock-scrambled), pBabe Hygro and pLKO.1-puro-TRF1 shRNA (mock-shTRF1), pMXs-Klf4, pMXs-Sox2, pMXs-Oct3/4 and pLKO.1-puro-scramble shRNA (3F-scramble), pMXs-Klf4, pMXs-Sox2, pMXs-Oct3/4 and pLKO.1-puro-TRF1 shRNA (3F-shTRF1). The procedure was repeated every 12 h for 2 days (a total of four additions). After infection was completed, media was replaced with standard ES media supplemented with KSR (Invitrogen) and with puromycin to select for the shRNAs vectors. Cultures were maintained in the presence of drug selection with daily medium changes. Reprogramming was assessed 2 weeks post infection by counting alkaline phosphatase-positive colonies. Alkaline phosphatase staining was performed according to manufacturerŕs instructions (BCIP/NBT Color Development Substrate, Promega). The results were normalized to the respective efficiencies of retroviral transduction as assessed by transducing with the three pMXs-Oct3/4, pMXs-Klf4 and pMXs-Sox2 retroviruses plus a retrovirus expressing GFP. Conditional TRF1 ablation in the small intestine Seven to 9-week old TRF1 lox/lox ; Villin-CreERT2 +/T mice and control TRF1 lox/lox ; Villin-CreERT2 +/T mice (C57BL/6) were injected intraperitonealy with 1 mg 4-OHT (Sigma) dissolved (with sonication) in 100 μl corn oil (Sigma-Aldrich). Injections were perfomed on a daily base (for 34 days). Mouse weight was measured every day. Two TRF1 lox/lox ; Villin-CreERT2 +/T mice had to be killed before day 34 owing to severe weight loss. Of all the mice, the intestines were extracted and prepared for western blot analysis, DNA-extraction and paraffin embedding after fixation over night with formalin. How to cite this article: Schneider, R. P. et al . TRF1 is a stem cell marker and is essential for the generation of induced pluripotent stem cells. Nat. Commun. 4:1946 doi: 10.1038/ncomms2946 (2013).